Optophononics with coupled quantum dots Modern technology is founded on the intimate understanding of how to utilize and control electrons. Next to electrons, nature uses phonons, quantized vibrations of an elastic structure, to carry energy, momentum and even information through solids. Phonons permeate the crystalline components of modern technology, yet in terms of technological utilization phonons are far from being on par with electrons. Here we demonstrate how phonons can be employed to render a single quantum dot pair optically transparent. This phonon-induced transparency is realized via the formation of a molecular polaron, the result of a Fano-type quantum interference, which proves that we have accomplished making typically incoherent and dissipative phonons behave in a coherent and non-dissipative manner. We find the transparency to be widely tunable by electronic and optical means. Thereby we show amplification of weakest coupling channels. We further outline the molecular polaron’s potential as a control element in phononic circuitry architecture. Phonons are central to the emerging technology termed ‘phononics’ [1] , [2] , [3] . Associated mainly with heat, lost energy and noise, phonons are encountered as such in many devices used in daily life. They also govern fundamental phenomena at the quantum level, from relaxation dynamics in nanostructures [4] , [5] , [6] , [7] , state broadening [8] to superconductivity [9] . In the development of solid-state quantum technologies, phonons are mainly considered for the limitations they impose. Omnipresent electron–phonon interactions and the predominantly dissipative nature of phonons are a major source of decoherence of the atom-like quantum states hosted by low-dimensional solid-state structures, such as quantum dots (QDs) [10] , [11] , [12] . A growing interest in coherent phonons in nanostructured materials marks a development that is beginning to utilize phonons as a technological resource that goes beyond that of a tool for spectroscopy [13] , [14] , [15] , [16] , [17] , [18] . QDs and quantum dot molecules (QDMs) are being intensely studied as controllable interfaces of charge, spin and photonic quantum states at the single particle level [19] , [20] , [21] , [22] , [23] . Phonons are recently beginning to enter this realm of mutual control of individual quantum states as mediators of the coupling of QDs to photonic cavity modes [24] , [25] . Already much gainful use of phonons is being made on a different scale, namely, in optomechanics [26] , [27] . Therein, the phonons’ attraction stems from the complementary nature of photons and phonons with regard to quantum information, with photons as broad band long-distance information carriers and phonons as long-time information storage. In epitaxial structures, phonons could take on both roles, provided they can be controllably utilized. We report a mechanism by which these phonons are made non-dissipative and coherent via electric field control and the optically driven formation of a molecular polaron in a pair of QDs. The concept of a polaron was first introduced by Landau as a quasi-particle formed by a charge and the deformation of the lattice it causes [28] . Particularly favourable are resonant polaron states as they can exhibit very long coherence times [29] , [30] , [31] . Here, a novel resonant polaron, a molecular polaron in a QDM, is being introduced. An induced optical transparency, the result of a Fano-type [32] , [33] resonant quantum interference, reveals the molecular polaron and its coherent nature [34] , [35] . We demonstrate the molecular polarons’ applicability as an amplifier of the visibility of weakest tunnel coupling channels. This observation via destructive interference proves the molecular polarons’ ability to make typically incoherent and dissipative phonons behave in a coherent and non-dissipative manner, thereby enhancing coherent interaction between two dots. Exciton and polaron transitions in QDMs We use QDMs formed by two vertically stacked self-assembled InAs/GaAs QDs [36] . The QDs are separated by a 4 nm GaAs barrier and embedded in an electric field effect structure. Both QDs forming a QDM possess the discrete, atom-like energy spectrum of single QDs. The molecular character of a QD pair is most clearly revealed in form of avoided crossings of the dots’ spectrally sharp optical transition lines in an electric field-dispersed optical spectrum of the QDM [36] , [37] , [38] , [39] . An electric field along the QDM axis shifts the energy levels of both dots overall and with respect to each other, shifting charges between and in and out of the QDM ( Fig. 1a,b ). 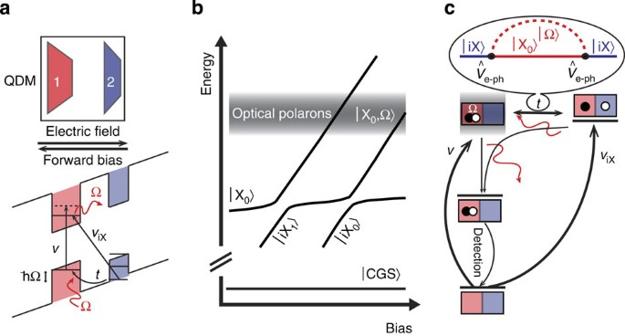Figure 1: Fano effect and molecular polaron formation. (a) Quantum dot molecule (QDM) sample geometry and band diagram indicating the optical,νandνiX, electronic,t, and phononic processes, Ω. (b) Schematic electric field-dispersed spectrum of a molecular neutral exciton showing the single QD-like ground-state exciton in QD1, |X0, its first optical polaron band, |X0,Ωand interdot excitons, |iXn, with the hole in thenth excited-state level of QD2. (c) Energy level diagram for an electric field where a Fano-like resonance between |iXand |X0,Ωcreates a molecular polaron, (|iX±|X0,Ω). Top: Feynman diagram describing the formation of the molecular polaron and producing the self-energyΣph(ω) in the optical Green functionG(ω) (equation 1). Figure 1: Fano effect and molecular polaron formation. ( a ) Quantum dot molecule (QDM) sample geometry and band diagram indicating the optical, ν and ν iX , electronic, t , and phononic processes, Ω. ( b ) Schematic electric field-dispersed spectrum of a molecular neutral exciton showing the single QD-like ground-state exciton in QD1, |X 0 , its first optical polaron band, |X 0 ,Ω and interdot excitons, |iX n , with the hole in the n th excited-state level of QD2. ( c ) Energy level diagram for an electric field where a Fano-like resonance between |iX and |X 0 ,Ω creates a molecular polaron, (|iX ±|X 0 ,Ω ). Top: Feynman diagram describing the formation of the molecular polaron and producing the self-energy Σ ph ( ω ) in the optical Green function G (ω) (equation 1). Full size image For clarity and without loss of generality, we limit the discussion to neutral excitons with their electron located in the ground state of the lower band-gap dot (here QD1) of the QDM; the hole may be in either dot and any state. Figure 1b schematically depicts the electric field-dispersed energy spectrum of a neutral exciton in a QDM. All states are labelled in terms of the type of exciton, |X n for a single QD-like exciton with electron and hole in the same dot (here QD1), or |iX n for an interdot exciton with the hole in the other QD than the electron (QD2). The index n is used to indicate the number of the hole level in the respective dot, where ‘0’ refers to the ground-state level and ‘ n >0’ to the n th excited-state level ( Fig. 1b ). The |X n states exhibit weak electric field dependence. The |iX n states exhibit much larger electric field dependence owing to the greater spatial separation of the charges and the resulting larger electric dipole moment [36] . This large dipole moment allows us to easily tune the interdot exciton states into resonance with states consisting of the |X 0 exciton and one optical phonon, labelled |X 0 ,Ω , which for InAs/GaAs-QDs are between 28 and 38 meV above the involved exciton state. These exciton-phonon states, so-called polarons, are continuous because of the k-space dispersion of the optical phonons, strain, intermixing of InAs and GaAs, and interface effects [40] , [41] . Optical transitions between all those states and the crystal ground state, |cgs , map the level structure of a QDM one to one into the optical spectrum. An overview optical spectrum of the example QDM to be discussed in the following can be seen in Supplementary Fig. 1 . Phonon-induced Fano effect in QDMs A Fano-like configuration of the energy levels is obtained when the energy difference between the ground-state hole level in QD1 and the n th hole level in QD2 matches the energy quantum, ħΩ, carried by an optical phonon ( Fig. 1a ). In this case, the n th interdot exciton state, |iX n , is in resonance with the continuum of optical polaron states, |X 0 ,Ω ( Fig. 1b,c ). A Fano effect will be observed only if coupling, t , exists between both states, causing interference between the two optical pathways, ν and ν iX ( Fig. 1c ). Thus, the observation of the Fano effect reveals a coupling channel [42] . Vice versa , the optical excitation of the system in this configuration induces an interaction between the QDs by enabling the QDs to couple via the interdot exciton and polaron states and the formation of a molecular polaron, |MP =|iX n ±|X 0 ,Ω ( Fig. 1c ). In the following, we verify this phonon-induced Fano effect and demonstrate the molecular polaron and its characteristics as an optophononic transparency. Similar in nature, resonant polaron states were described for the regime of cyclotron resonance [29] , [31] and in multiquantum wells [30] . Here we employ a simplified model to simulate the optical absorption of the QDM. The energy absorption rate of our system can be calculated using the diagrammatic technique ( Fig. 1c ; Supplementary Note 1 and Supplementary Figs 2–4 ). Selecting one resonant quantum state |iX n ( Fig. 1 ), we obtain the absorption spectrum from where and are the transition energies of the corresponding excitons, V g is a gate voltage, Δ ph =π ρ 0 t 2 is the phonon-assisted tunnelling broadening, ρ 0 is the phonon density of states, is the Fano factor; ω ph,0 and D are the central phonon energy and a half-width of the phononic band. The self-energy is a result of the coherent coupling between the electron in the valence band of a QDM and the phonon modes. Equation (1) is reduced to the original Fano formula in the limit D →∞. The sign of q Fano depends on the product of signs of the two quantum amplitudes ν and ν iX . This is a characteristic feature of a quantum interference effect. When >> 1 the Fano effect is weak and the line is symmetric, when the line becomes strongly asymmetric and when the spectrum typically shows an anti-resonance (dip), that is, a narrow transparency window. The asymmetry of the absorption structures is a result of the interference in the Fano scheme ( Fig. 1c ) and is controlled by the parameter . The spectrum will also depend on the relative position of the photon energy in the phonon band. The calculated grey-scale plot in Fig. 2a illustrates the theoretically expected features of a Fano resonance with q =1. Similar features are found in the experimental data where interdot exciton transitions traverse the optical phonon bands, as seen in Fig. 2b for the optical transition into the |iX 4 of an example QDM. Line cuts extracted from the electric field-dispersed spectrum in Fig. 2b reveal derivative and anti-resonance-like line shapes that are typical for a Fano effect with a positive q -factor ( Fig. 2c–h ). We also find experimental examples of Fano resonances with any other possible value of q Fano , including q Fano ≈0 (not shown) and q Fano <0 ( Fig. 2i–n ). Additional validation of the phonon-based Fano scheme is obtained through an analysis of the Fano factor, which yields ν ≈20 ν iX –300 ν iX and interdot exciton lifetimes on the order of a few ten to a few hundred nanoseconds in agreement with recent experiments [43] (see Supplementary Note 2 ). This analysis proves that the Fano effect with phonons is the mechanism underlying the optical transparency, and demonstrates that QDMs provide a system in which this induced optical transparency is widely tunable. 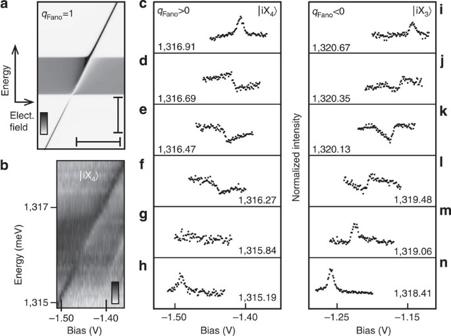Figure 2: Phonon-induced transparency. (a) Theoretical and (b) experimental examples of Fano resonances. The theoretical example was calculated withqFano=1. The intensity in the experimental data was normalized to the maximum signal at each energy step. Scale bars, 1 meV and 0.1 V (a). The grey-scale indicates absorption (PLE intensity), with darker meaning stronger absorption. (c–h) Line cuts extracted from the experimental example inashowing Fano line shapes characteristic of a positive Fano factor (qFano≈+1) as the transition into |iX4of a QDM traverses an optical polaron band. (i–n) Fano line shapes characteristic of a negative Fano factor (qFano≈−1) as the transition into |iX3of the same QDM as inbandc–htraverses a different optical polaron band. The spectra inc–handd–nwere normalized to the difference between minimum and maximum signal. A signal decrease to about 60% of the maximum signal is the maximum transparency observed in the two data sets shown (panelseandk). The numbers in the bottom of each panel indicate the laser excitation energy at which the respective spectrum was obtained. An overview spectrum of the studied molecule is shown inSupplementary Fig. 1. Figure 2: Phonon-induced transparency. ( a ) Theoretical and ( b ) experimental examples of Fano resonances. The theoretical example was calculated with q Fano =1. The intensity in the experimental data was normalized to the maximum signal at each energy step. Scale bars, 1 meV and 0.1 V ( a ). The grey-scale indicates absorption (PLE intensity), with darker meaning stronger absorption. ( c – h ) Line cuts extracted from the experimental example in a showing Fano line shapes characteristic of a positive Fano factor ( q Fano ≈+1) as the transition into |iX 4 of a QDM traverses an optical polaron band. ( i – n ) Fano line shapes characteristic of a negative Fano factor ( q Fano ≈−1) as the transition into |iX 3 of the same QDM as in b and c – h traverses a different optical polaron band. The spectra in c – h and d – n were normalized to the difference between minimum and maximum signal. A signal decrease to about 60% of the maximum signal is the maximum transparency observed in the two data sets shown (panels e and k ). The numbers in the bottom of each panel indicate the laser excitation energy at which the respective spectrum was obtained. An overview spectrum of the studied molecule is shown in Supplementary Fig. 1 . Full size image The q -factor clearly affects the character of the molecular polaron as an induced optical transparency. Different q -factors can be realized with different molecular polarons. Alternatively, nonlinearities in the Fano effect [42] may provide a tuning mechanism of the transparency window. 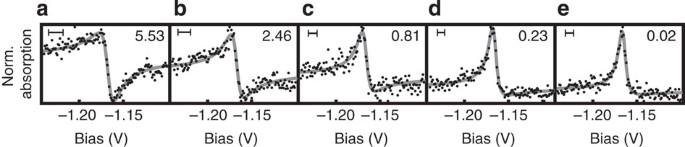Figure 3: Nonlinearity of the phonon-induced Fano effect. (a–e) Excitation power dependence of the Fano line shape at power densities in nW μm−2as indicated in the top right corner of each panel. The solid lines are fits to the data according to equation (1). Scale bars indicate the full width at half maximum. Figure 3a–e examines the power dependence of the line shape of the transition into |iX 4 at an excitation energy of 1,322 meV (ħ Ω =35 meV). At low powers the line shape is nearly Lorentzian. As the power increases, the line shape evolves from Lorentzian via a derivative-like phase to anti-resonance-like, confirming tunability of the optical transparency. From the detailed analysis of the power dependence, we find the underlying mechanism to be an increase of the phonon-mediated tunnel coupling, t , between the two states ( Supplementary Note 3 and Supplementary Fig. 5 ). Figure 3: Nonlinearity of the phonon-induced Fano effect. ( a – e ) Excitation power dependence of the Fano line shape at power densities in nW μm −2 as indicated in the top right corner of each panel. The solid lines are fits to the data according to equation (1). Scale bars indicate the full width at half maximum. Full size image Note that one can attribute each individual dot a marginal phonon confinement with an excellent bulk-phonon approximation for the nature of the phonons. The formation of a molecular polaron drastically changes the nature of the phonon. In the single QD-like polaron state |X 0 ,Ω , the bulk-like nature of the phonon dominates the state—volatile, dissipative and of very short coherence. Coherent coupling to an interdot exciton state |iX n traps the phonon in the QDM system and makes it long lived. The optical transparency is the manifestation of this process of an optically driven and electrically tunable localization of phonons, that is, not only does the mechanical excitation of the system influence the electronic QDM states, but the electronic QDM states also strongly influence the mechanical excitation. With the formation of a molecular polaron in a pair of QDs, we demonstrate how bulk-like phonons can be localized and therefore made technologically usable with the ease of an electric field control. Applications of the molecular polaron As a consequence of an amplified coupling, interdot transitions should exhibit a similar enhanced visibility, which we verify in Fig. 4a–c . Note how the transition into |iX 3 is, if at all, barely visible outside the phonon band, yet reduces the signal of the phonon band by about 75%. This observation proves that the interference signal is caused not just by additive or subtractive superposition of the two paths’ amplitudes, but also by amplification. One may think of the nonlinear process as two oscillators being synchronized by the optical driving field, which would imply an increase in coherence of the coupling. In fact, while an enhanced signal looking like constructive interference may just be an increased absorption cross-section and incoherent coupling of the involved states, destructive interference signals demand coherence between the states. In this sense, the molecular polaron can be used as an efficient and tunable coherent coupler for quantum states in spatially separated low-dimensional structures. 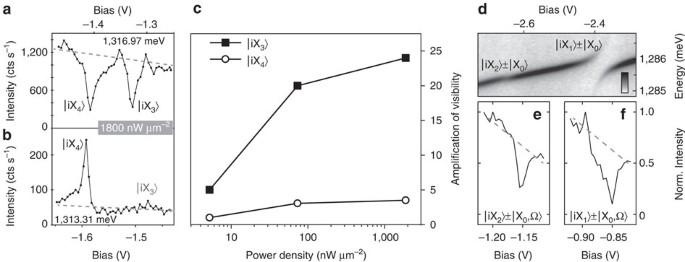Figure 4: Fano amplification effect. PLE intensity profiles of the interdot transitions into the states |iX3and |iX4at excitation energies in (1,316.97 meV, (a)) and off (1,313.31 meV, (b)) resonance with the phonon band. (c) Signal ratios of the transitions into the two states at excitation energies on and off resonance with the phonon band as a function of excitation power. For the signal of the transition into |iX3, a lower limit of the amplification was calculated using the full width of the noise. (d) Electric field-dispersed PL spectrum of the |X0state showing the anticrossings caused by hole level resonances with the interdot excitons |iX1and |iX2with tunnelling rates,t1=0.36 meV andt2=0.06 meV. The grey scale indicates PL intensity, with darker meaning higher intensity. (e,f) The phonon-induced transparency signal caused by the phonon-mediated hole tunnelling between the same single QD-like exciton state and the interdot exciton states as ind. The dashed lines indicate the base line to which the signal (dip or peak) is referenced to. Figure 4: Fano amplification effect. PLE intensity profiles of the interdot transitions into the states |iX 3 and |iX 4 at excitation energies in (1,316.97 meV, ( a )) and off (1,313.31 meV, ( b )) resonance with the phonon band. ( c ) Signal ratios of the transitions into the two states at excitation energies on and off resonance with the phonon band as a function of excitation power. For the signal of the transition into |iX 3 , a lower limit of the amplification was calculated using the full width of the noise. ( d ) Electric field-dispersed PL spectrum of the |X 0 state showing the anticrossings caused by hole level resonances with the interdot excitons |iX 1 and |iX 2 with tunnelling rates, t 1 =0.36 meV and t 2 =0.06 meV. The grey scale indicates PL intensity, with darker meaning higher intensity. ( e , f ) The phonon-induced transparency signal caused by the phonon-mediated hole tunnelling between the same single QD-like exciton state and the interdot exciton states as in d . The dashed lines indicate the base line to which the signal (dip or peak) is referenced to. Full size image The molecular polaron’s power as a tunable coherent coupler can be seen as follows. In Fig. 4d–f we compare the two tunnel resonances of the single QD-like exciton ground state, (|iX 1 ±|X 0 ) and (|iX 2 ±|X 0 ), with the corresponding two molecular polaron resonances, (|iX 1 ±|X 0 ,Ω ) and (|iX 2 ±|X 0 ,Ω ). The tunnelling rates of the two resonances with the bare single QD-like exciton are vastly different, with (355±20) μeV and (65±25) μeV ( Fig. 4d ). In contrast, the molecular polaron resonances are of nearly identical transparency ( Fig. 4e,f ). From the large visibility achieved here it follows that even much weaker coupling channels can be boosted this way, and thus also coupling over larger distances. While the dot separation accessible for quantum mechanical tunnel coupling may be boosted to the 100 nm range, as the amplification and off resonance residual coupling strength suggest (see Supplementary Note 4 and Supplementary Fig. 6 ), transfer of the molecular polaron concept to other coupling mechanisms, such as radiative coupling, has the potential to bridge even larger distances. Unlike discrete excited electronic states, the optical polaron states have a well-defined energy difference to the ground state, turning the phonon-induced transparency into a predictable and reliable tool for revealing small coupling channels and making them usable. A future application of the molecular polaron can be derived from the fact that the underlying fundamental mechanism of the phonon-induced optical transparency, the Fano effect, does not rely on the optical excitation as employed here. The three critical elements of the Fano effect are two energetically degenerate states of which one is discrete and the other is a continuum state, the existence of coupling between both states and the resonant transition from a common state into the two energetically degenerate states. Thus, the reversal of our experiment, that is, the interaction of a phonon with a pre-existing electronic state, , can result in an optically induced phonon transparency. Together with phononic crystal waveguides [1] , phononic leads that allow for a flow of suitable phonons through the QDM, the molecular polaron has the potential to serve as an electric field-driven control element for the flow of phonons. In contrast to previous concepts [44] , [45] such an all solid-state design can be integrated with conventional nanotechnology integrated circuitry architectures. The above discussion reveals that phonons can be made to interact in a coherent manner with photons and charges in coupled QDs through the formation of a molecular polaron. The revealed mechanism to localize phonons via electric field control provides fresh possibilities for phononics and quantum technologies, especially as metastable electronic ground states may be utilized. We have outlined how the molecular polaron can act as a control element in phononic circuits. As such, the molecular polaron can be utilized in phase-coherent information transfer between coupled QDs embedded in phononic crystal waveguide structures. In phononic cavities, coherent coupling of electronic states of two QDMs, A and B, could be achieved, such as ( c 1 |X 0 ,Ω A |iX n B ± c 2 |iX n A |X 0 ,Ω B ). In combination with photonic structures, a device architecture can be envisioned where photons are used for interlayer (vertical) and phonons for intralayer (lateral) quantum information transfer and processing, with QDMs as interfaces between the channels. Room temperature applications of the phonon-induced transparency are conceivable by transferring the concept to other coupled atom-like solid-state structures, such as coupled nitrogen-vacancy centres in diamond. Samples The QDMs used in this study were fabricated by molecular beam epitaxy. Embedded in the intrinsic region of a Schottky diode structure, the two layers of QDs were formed by subsequent deposition of InAs on GaAs with a 4 nm thick barrier of GaAs between both layers. The full sequence of layers deposited on top of the GaAs substrate was 500 nm n + -GaAs buffer, 80 nm i-GaAs, 2.5 nm InAs QDs, 4 nm GaAs barrier, 2.5 nm InAs QDs, 230 nm GaAs, 40 nm Al 0.3 Ga 0.7 As, 10 nm GaAs, 8 nm titanium and 120 nm aluminium. The aluminium layer contained micrometre-sized apertures for optical access. The sample was mounted and electrically contacted in a ceramic chip header. The dot layers were grown with density gradients by interrupting the wafer rotation during the respective molecular beam epitaxy growth steps. The density of QDs in the region of the wafer where the studied sample was taken from was between 10 8 and 10 9 cm −2 . The heights of the dots were adjusted by the so-called indium flush technique. For this technique the capping of the dots with GaAs is interrupted at a layer thickness that defines the desired height. Then, the temperature is raised allowing the exposed InAs to redistribute and evaporate before the regular growth of the GaAs barrier is continued. The height of dots in both layers was nominally set to 2.5 nm. Dots in the second layer were found to exhibit higher band gaps than dots in the first layer, which is attributed to a larger lateral growth of dots in the second layer causing a different evolution of the dots during the indium flush [46] , [47] , [48] . Experiment The samples were mounted on the cold finger of a closed cycle microscopy cryostat and kept at a temperature of 20 K. A tunable diode laser with a tuning range from about 900 to 1,000 nm and a line width of <300 kHz was used for photoluminescence (PL) experiments at a wavelength of 918 nm and for photoluminescence excitation (PLE) experiments across the wavelengths (energies) specified in the figures. The QD photoluminescence was spectrally dispersed in the third stage of a triple spectrometer by a 1,100-cm −1 line grating and detected with a liquid nitrogen-cooled charge-coupled device camera. The first two stages of the spectrometer were used in subtractive mode as a high-quality band pass filter to suppress scattered laser light. Additional long and short pass filters were used in the detection and excitation paths, respectively. The electric field-dispersed PLE spectra were composed from electric field-dispersed PL spectra taken at different laser excitation energies by summing the intensity of the PL transition |X 0 →|cgs over a narrow spectral range centred about the maximum intensity of this transition at each field step. For this study, detailed PLE measurements were performed on three QDMs from the sample with 4 nm barrier, all showing phonon-induced optical transparency. The data presented here are from one example molecule. In addition, the effect was also verified in a sample with QDMs with a 6-nm barrier. Electric field-dependent PLE spectra such as seen in Fig. 2b and Supplementary Fig. 1A are composed of about eight energy steps per meV. Data analysis The fits of the data in Fig. 4 to equation (1) were performed in the following way. The relative position of the photon energy in the phonon band was determined from electric field-dispersed PLE spectra such as ( Supplementary Fig. 1 ). An offset was included in equation (1) to rescale the data so that the Fano minimum equals zero and the polaron background one. How to cite this article: Kerfoot, M. L. et al. Optophononics with coupled quantum dots. Nat. Commun. 5:3299 doi: 10.1038/ncomms4299 (2014).